A pervasive role for biomass burning in tropical high ozone/low water structures Air parcels with mixing ratios of high O 3 and low H 2 O (HOLW) are common features in the tropical western Pacific (TWP) mid-troposphere (300–700 hPa). Here, using data collected during aircraft sampling of the TWP in winter 2014, we find strong, positive correlations of O 3 with multiple biomass burning tracers in these HOLW structures. Ozone levels in these structures are about a factor of three larger than background. Models, satellite data and aircraft observations are used to show fires in tropical Africa and Southeast Asia are the dominant source of high O 3 and that low H 2 O results from large-scale descent within the tropical troposphere. Previous explanations that attribute HOLW structures to transport from the stratosphere or mid-latitude troposphere are inconsistent with our observations. This study suggest a larger role for biomass burning in the radiative forcing of climate in the remote TWP than is commonly appreciated. Tropospheric O 3 is an important greenhouse gas. Ozone has exerted an increase in the global radiative forcing of climate of ∼ 0.4 Wm −2 between 1750 and 2011, almost equal to that of CH 4 over the same time period [1] . The largest contribution to the climatic influence of O 3 is due to enhancements over background in the tropical troposphere [2] , [3] . Elevated surface O 3 adversely affects human health and agriculture [4] , [5] . Legislation enacted to protect public health has significantly reduced emissions of O 3 precursors from automobiles, factories and power plants throughout the industrialized world, particularly in the Northern Hemisphere mid-latitudes [6] , [7] . Surface O 3 levels in the industrialized extra-tropics have plateaued or fallen dramatically in response to these actions [8] , [9] . It is unclear whether the measures taken to reduce surface O 3 in the extra-tropics will reduce the climatic impact of O 3 , since its largest radiative influence is in the tropics. In the marine boundary layer (MBL) of the tropical western Pacific (TWP), O 3 is removed by photochemical reactions involving halogen radicals of marine biogenic origin, resulting in O 3 abundances of ∼ 20 p.p.b.v. or lower [10] , [11] . Local convection can transmit this low O 3 air throughout the tropospheric column [12] , resulting at times in O 3 profiles that have mixing ratios of ∼ 20 p.p.b.v. over an extended altitude range [13] , [14] . Air masses with elevated O 3 are frequently accompanied by water vapour mixing ratios depressed with respect to the local background, particularly in the mid-troposphere [15] . These high ozone/low water (HOLW) structures inhibit mixing and convection [16] , alter the local radiative heating profile [17] , and affect the atmosphere’s oxidative capacity [13] . Large increases in O 3 relative to these low background values have frequently been observed in the TWP mid-troposphere [12] , [14] , [18] , [19] , [20] , [21] , [22] , [23] , [24] , [25] . Many of these studies note that water vapour tends to be depressed, with respect to the local background, for these high O 3 air parcels [12] , [14] , [18] , [19] , [20] , [21] , [22] , [24] , often attributing the HOLW structures to sources outside the tropical troposphere. Stoller et al . [19] conclude that stratospheric air is the dominant source of HOLW air parcels observed over the TWP during multiple aircraft campaigns conducted in September and October 1991, February and March 1994 and September and October 1996. This conclusion was mainly based on the co-location of high potential vorticity (PV) with a few HOLW structures. These early campaigns lacked the instrumentation to measure the suite of chemical compounds sampled during modern campaigns, particularly the biomass burning tracer HCN. Newell et al . [18] reach a similar conclusion, analysing the same data as Stoller et al . in addition to observations from the MOZAIC campaign from between 1994 and 1997. They note elevated CO and CH 4 in some of their observed HOLW structures, citing entrainment of biomass burning emissions into stratospheric air. Using back trajectory analysis in addition to sonde measurements of O 3 and H 2 O from 6 years of Southern Hemisphere ADditional OZonesonde Experiment (SHADOZ) data at three Pacific sites, Hayashi et al . [20] argue that transport from the mid-latitude upper troposphere (mlUT) is the dominant source of high mid-tropospheric O 3 in the TWP, with biomass burning only a minor contributor in some months. Kley et al . [12] likewise hypothesize a mlUT origin for HOLW features near 700 hPa measured by ozonesondes in the equatorial western Pacific during the CEPEX and TOGA-COARE campaigns conducted during fall 1992. Finally, Ridder et al . [25] attribute enhancements in O 3 and CO observed remotely in the Northern Hemisphere TWP during October and November 2009 to fossil fuel combustion in Asia, Europe and North America (that is, the mid-latitudes) and in the Southern Hemisphere (SH) to both fossil fuel combustion and biomass burning. Numerous other studies claim that low H 2 O in the TWP mid-troposphere, defined here as 300–700 hPa, is dominated by the transport of dry air from the mid-latitudes. Yoneyama and Parsons [26] conclude horizontal advection from the mid-latitudes, likely through Rossby wave breaking, creates the observed distribution of dry air during the TOGA-COARE experiment. Combining satellite data and trajectory simulations, Waugh [27] finds that high PV intrusions in the subtropics lead to low relative humidity (RH) in the intrusion itself and high RH ahead of the intrusion, consistent with transport from the lower stratosphere and the deep tropical troposphere, respectively. Cau et al . [28] conclude that a dominant dry air source in the TWP is dehydration of air parcels via poleward movement of tropical, upper tropospheric air into the jet followed by slow descent driven by radiative cooling. This study relied on 24-day back trajectories and did not account for the presence of convective precipitation, which is known to greatly alter air mass composition. Galewsky et al . [29] conclude, using a tagged tracer method and reanalysis data, that mid-latitude eddies and isentropic transport are the dominant source of low H 2 O in the subtropics in December–February 2001/2002. This analysis focused on the zonal mean distribution of H 2 O. The subtropical location of their water minimum is coincident with earth’s major deserts, which means this region is decoupled from convective precipitation that rehydrates other regions of the tropics. Conversely, Dessler and Minschwaner [30] concluded that deep convective outflow associated with the Hadley circulation is the largest source of low H 2 O in the tropical eastern Pacific. Our analysis, which focuses on the tropics (20° N–20° S) of the western Pacific, similarly suggests low water is controlled by outflow of the Hadley circulation. Other studies cite the importance of biomass burning in controlling tropical O 3 , particularly over the Atlantic Ocean and in the SH, but fail to account for the origin of low H 2 O in HOLW air parcels. Jacob et al . [31] find that tropical processes alone, including in situ photochemical production from biomass burning emissions and lightning NO x (NO x =NO+NO 2 ), can reproduce observed tropical O 3 distributions using measurements over the South Atlantic during the TRACE-A campaign in September and October 1992. Other studies have attributed high O 3 observed in the TWP to photochemical production in biomass burning plumes. Oltmans et al . [14] investigated the O 3 climatology over three locations (Fiji, Samoa and Tahiti) in the TWP from the SHADOZ network. Elevated, mid-tropospheric O 3 was found at these sites, particularly in September and October. Back trajectory analysis connected some of these O 3 enhancements in Fiji and Samoa to biomass burning in Indonesia, and it was noted that air parcels descended ∼ 3 km in transit. In the PEM-Tropics A mission conducted in the Eastern and Central Pacific of the SH in August and September 1996, both Blake et al . [21] and Singh et al . [22] attribute elevated O 3 in HOLW parcels to photochemical production from biomass burning in Africa and South America based on elevated mixing ratios of biomass burning tracers (C 2 H 2 , NO x , CO, CH 3 Cl, PAN and C 2 H 6 ) in the structures. Similar to Oltmans et al ., Blake et al . and Singh et al . posit large-scale subsidence as a possible cause of the low H 2 O but offer no quantitative support for this supposition. Folkins et al . [24] observed HOLW air over Fiji (18° S) at ∼ 120 hPa during the ASHOE/MAESA campaign in October 1994. These air parcels were enhanced in reactive nitrogen compounds and had high N 2 O mixing ratios, indicative of a tropospheric origin. They attributed the low H 2 O to transport from the mlUT using 10-day isentropic trajectories but did not provide any quantitative analysis of the effect of thermodynamics or descent on observed H 2 O. Finally, Kondo et al . [23] attribute increases in O 3 of 26 p.p.b.v. over a 31 p.p.b.v. background in the western Pacific to biomass burning during the TRACE-P campaign (February–April 2001). These studies either ignore the low H 2 O (ref. 23 ), offer limited explanation [14] , [21] , [22] , attribute low H 2 O to extra-tropical transport [24] , or do not describe H 2 O (ref. 31 ). The source of high O 3 as well as the dynamical processes controlling the low H 2 O in HOLW structures prevalent in the TWP is clearly unresolved. Here we analyse aircraft and ozonesonde observations, model output, and satellite data to understand the origin of the HOLW air parcels observed in the TWP during winter 2014. The Coordinated Airborne Studies in the Tropics (CAST) and CONvective TRansport of Active Species in the Tropics (CONTRAST) aircraft campaigns based in Guam (13.5° N, 144.8° E) provide a comprehensive suite of chemical measurements. We examine the 17 CAST and 11 CONTRAST flights that provided unprecedented sampling of the TWP mid-troposphere during January and February 2014 ( Fig. 1 ). These in situ observations are supplemented by satellite measurements of water vapour and outgoing longwave radiation (OLR) from the daily Atmospheric Infrared Sounder (AIRS) product as well as fire counts from the Moderate Resolution Imaging Spectroradiometer (MODIS) instrument. Ten day, kinematic back trajectories were initialized along the CAST and CONTRAST flight tracks using the Hybrid Single Particle Lagrangian Integrated Trajectory (HYSPLIT) model to connect observed air parcels to their source regions. The CAM-Chem chemical transport model was run with tagged biomass burning tracers to further elucidate ozone sources and was evaluated with ozonesonde observations from the SHADOZ network. Models, satellite data and aircraft observations are used to show that anthropogenic fires in tropical Africa and Southeast Asia are the dominant source of the high O 3 and that the low H 2 O results from large-scale descent within the tropical troposphere, after detrainment of biomass burning plumes. 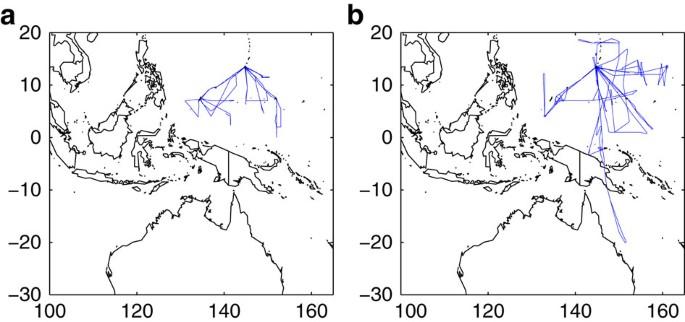Figure 1: Flight tracks for the CAST and CONTRAST campaigns. Tracks for (a) CAST and (b) CONTRAST flights analysed in this study. Figure 1: Flight tracks for the CAST and CONTRAST campaigns. Tracks for ( a ) CAST and ( b ) CONTRAST flights analysed in this study. Full size image Source of high ozone in the TWP Representative O 3 , CO and H 2 O profiles from the CAST and CONTRAST campaigns are shown in Fig. 2 . Unless otherwise specified, all references to H 2 O in this paper refer to water vapour observations from an open-path laser hygrometer with complete discrimination against condensed water [32] . Mixing ratios of O 3 and H 2 O in these profiles exhibit strong anti-correlation; that is, elevated O 3 is closely associated with low RH [15] . These HOLW structures were a pervasive feature seen throughout both campaigns. Here we define a HOLW structure as an air parcel satisfying the simultaneous criteria of O 3 >40 p.p.b.v. and RH <20%, where RH in this study is with respect to water for T>273 K and to ice for T<273 K. Relying solely on composition to define HOLW structures allows for the inclusion of both sharply defined, thin features (for example, Fig. 2a ) as well as those that occupy a large fraction of the tropospheric column (for example, Fig. 2d ). HOLW features were primarily located between 300 and 700 hPa and observed during 45 of 104 independent profiles (that is, air parcels were not intentionally resampled). For air parcels with RH >20%, median O 3 was nearly constant with altitude at ∼ 20 p.p.b.v. ( Fig. 3a ). For air with RH <20%, median O 3 peaked at 60 p.p.b.v. near 450 hPa, three times greater than background, and decreased to ∼ 40 p.p.b.v. at 750 and 300 hPa. 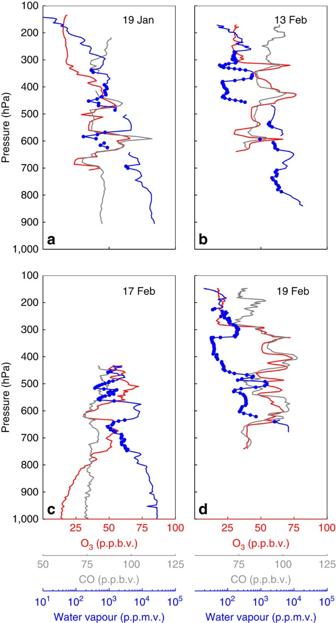Figure 2: Ozone, water vapour and CO profiles in the TWP. Sample profiles of 10 s averaged O3(red), CO (grey) and H2O (blue) from four flights during CONTRAST (a,b,d) and CAST (c). Blue circles indicate measurements of H2O mixing ratios for which RH <20%. RH is with respect to water and with respect to ice for temperatures above and below 273 K, respectively. Vertical profiles have a characteristic horizontal length of∼300 km. Figure 2: Ozone, water vapour and CO profiles in the TWP. Sample profiles of 10 s averaged O 3 (red), CO (grey) and H 2 O (blue) from four flights during CONTRAST ( a , b , d ) and CAST ( c ). Blue circles indicate measurements of H 2 O mixing ratios for which RH <20%. RH is with respect to water and with respect to ice for temperatures above and below 273 K, respectively. Vertical profiles have a characteristic horizontal length of ∼ 300 km. 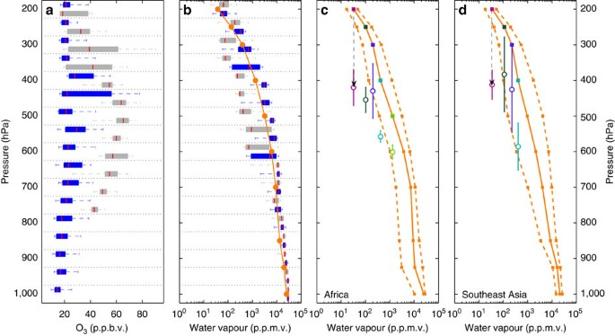Figure 3: Structure of ozone and water vapour in the TWP. (a) Profiles ofin situO3during CAST and CONTRAST for two modes of RH (blue, RH >20%; grey, RH <20%). Box and whisker plots show 5th, 25th, 50th, 75th and 95th percentiles for 50 hPa pressure bins. Each bin is delimited by a dotted line, and the two modes (grey and blue boxes) for a given pressure bin are offset for clarity. Between 400 and 700 hPa, the average (minimum) number of observations per blue and grey box is 650 (414) and 330 (43), respectively. Observations between 300 and 400 hPa were more limited with a minimum of 20 and a maximum of 56 observations. (b) Distribution of H2O for two modes of HCN (grey, HCN >150 p.p.t.v.; blue, HCN <150 p.p.t.v.). Median AIRS H2O over the ascending branch of the Hadley Cell (orange). Between 300 and 700 hPa, the average (minimum) number of observations per blue and grey box is 129 (28) and 111 (19), respectively. (c) Median (solid), 5th and 95th percentiles (dashed) of AIRS H2O over the African biomass burning region (orange). Open circles represent the mean end point of descent ±1σ of trajectories starting over the African biomass burning region and arriving over the TWP, for various initial pressures (closed squares).dSame ascbut for trajectories starting over Southeast Asia. Full size image Figure 3: Structure of ozone and water vapour in the TWP. ( a ) Profiles of in situ O 3 during CAST and CONTRAST for two modes of RH (blue, RH >20%; grey, RH <20%). Box and whisker plots show 5th, 25th, 50th, 75th and 95th percentiles for 50 hPa pressure bins. Each bin is delimited by a dotted line, and the two modes (grey and blue boxes) for a given pressure bin are offset for clarity. Between 400 and 700 hPa, the average (minimum) number of observations per blue and grey box is 650 (414) and 330 (43), respectively. Observations between 300 and 400 hPa were more limited with a minimum of 20 and a maximum of 56 observations. ( b ) Distribution of H 2 O for two modes of HCN (grey, HCN >150 p.p.t.v. ; blue, HCN <150 p.p.t.v.). Median AIRS H 2 O over the ascending branch of the Hadley Cell (orange). Between 300 and 700 hPa, the average (minimum) number of observations per blue and grey box is 129 (28) and 111 (19), respectively. ( c ) Median (solid), 5th and 95th percentiles (dashed) of AIRS H 2 O over the African biomass burning region (orange). Open circles represent the mean end point of descent ±1σ of trajectories starting over the African biomass burning region and arriving over the TWP, for various initial pressures (closed squares). d Same as c but for trajectories starting over Southeast Asia. Full size image Kinematic trajectories connect nearly all of these HOLW structures to tropical regions with active biomass burning. 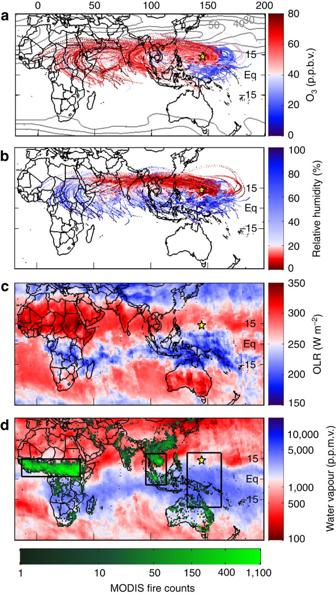Figure 4: Origins of air in the TWP. (a) 10-day, HYSPLIT back trajectories for all CAST flights analysed here and CONTRAST RF03–05 and RF07–14 for observed pressures between 300 and 700 hPa. Trajectories are stopped when encountering convective precipitation and coloured by observed O3. For clarity, only every third is shown. Contours are zonal winds at 200 hPa averaged over January and February 2014 in 10 m s−1intervals. The yellow star shows Guam.bSame asabut coloured by HYSPLIT RH along the trajectory (see methods). (c) AIRS daytime OLR averaged over CAST and CONTRAST flight days.dSame ascbut for AIRS H2O at 500 hPa. MODIS fire counts are the total for January and February 2014. Black rectangles represent the African and Southeast Asian tropical biomass burning regions (determined subjectively by the high fire counts) and the CAST/CONTRAST study region. Figure 4a,b shows 10-day back trajectories found using the HYSPLIT model [33] . Trajectories are coloured by observed aircraft O 3 (invariant along each trajectory) and RH along the trajectory as output by HYSPLIT (see Methods section). Each trajectory stops at our estimate of the point of last precipitating convection, derived from a combination of cloud top height and precipitation data from geostationary satellites and the Tropical Rainfall Measuring Mission satellite. We stop the trajectories at the point of last precipitating convection because convection lofts MBL air into the upper troposphere, where it detrains throughout the column, creating a nearly uniform O 3 profile and a water vapour profile controlled by the local saturation vapour pressure [15] . This convection effectively resets air parcel composition, removing any influence from outside the TWP. Further, global transport models are unable to reproduce the small-scale wind fields associated with deep convection, creating large uncertainty for back trajectories beyond this point. Air parcels originating from the clean SH and eastern Pacific had unimodal O 3 and RH distributions, with medians of 22 p.p.b.v. and 63%, respectively. Trajectories originating west of the study region, primarily over Africa and Southeast Asia, exhibit a bimodal distribution [15] . Assuming a mixture of two Gaussian distributions, the two modes are described by one with peak O 3 and RH of 21 p.p.b.v. and 60% and another with peaks of 55 p.p.b.v. and 4.5%. The low O 3 trajectories are indicative of air parcels under local influence (that is, convectively controlled in the TWP). The high O 3 trajectories originated over regions of active biomass burning in the tropics and reached the TWP along the upper branch of the Walker circulation ( Fig. 4a ). The rather substantial contribution of the HOLW structures to the overall atmospheric state of the TWP troposphere is quantified by Pan et al . [15] . Figure 4: Origins of air in the TWP. ( a ) 10-day, HYSPLIT back trajectories for all CAST flights analysed here and CONTRAST RF03–05 and RF07–14 for observed pressures between 300 and 700 hPa. Trajectories are stopped when encountering convective precipitation and coloured by observed O 3 . For clarity, only every third is shown. Contours are zonal winds at 200 hPa averaged over January and February 2014 in 10 m s −1 intervals. The yellow star shows Guam. b Same as a but coloured by HYSPLIT RH along the trajectory (see methods). ( c ) AIRS daytime OLR averaged over CAST and CONTRAST flight days. d Same as c but for AIRS H 2 O at 500 hPa. MODIS fire counts are the total for January and February 2014. Black rectangles represent the African and Southeast Asian tropical biomass burning regions (determined subjectively by the high fire counts) and the CAST/CONTRAST study region. Full size image Simultaneous elevation of CO and O 3 in the HOLW structures, in addition to regression analysis, suggests a tropospheric origin. Local maxima in O 3 and CO profiles closely track one another, with r 2 values between these two species ranging from 0.46 to 0.72 ( Fig. 5 ) for the profiles shown in Fig. 2 . A campaign-wide regression of CO and O 3 for air parcels that trace back to continental regions yields r 2 =0.61. Photochemical enhancement ratios of O 3 with respect to CO (ΔO 3 /ΔCO) for the profiles shown in Fig. 2 range between 0.97 and 2.85 mol mol −1 . Mauzerall et al . [34] found fresh biomass burning plumes had enhancement ratios of ∼ 0.15 mol mol −1 while plumes older than 6 days had values on the order of 0.75 mol mol −1 . These results are consistent with Parrington et al . [35] who found mean enhancement ratios of 0.81 mol mol −1 with a maximum ratio of 2.55 for boreal biomass burning plumes older than 5 days. Both comparisons suggest the air parcels analysed here are significantly aged and the enhancement ratios lie at the upper end of previous observations. This agrees with the back trajectories and photochemical aging analysis, discussed below, both of which yield air parcel ages of ∼ 10 days. NO is also elevated in these air parcels ( Supplementary Fig. 1 ), though the correlation with O 3 is not as prominent as for other species. This is likely due to the conversion of NO to other nitrogen-containing species, such as alkyl nitrates, peroxyacetyl nitrate and HNO 3 , none of which were measured during CAST and CONTRAST. 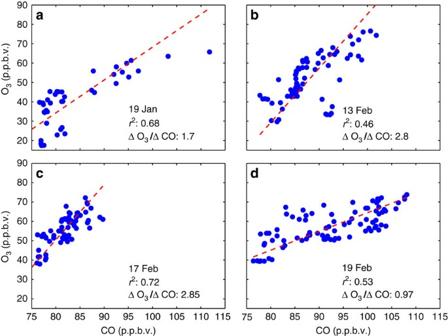Figure 5: Enhancement ratios of CO and ozone from CAST and CONTRAST. Regression of CO against O3for the data shown inFig. 2for pressures between 300 and 700 hPa (a–d). The ΔO3/ΔCO ratio for all profiles suggests significantly aged air, consistent with the back trajectory and photochemical aging analyses. The dashed red line is the best fit via orthogonal linear regression. Flight dates, slope andr2values are shown for all panels. Figure 5: Enhancement ratios of CO and ozone from CAST and CONTRAST. Regression of CO against O 3 for the data shown in Fig. 2 for pressures between 300 and 700 hPa ( a – d ). The ΔO 3 /ΔCO ratio for all profiles suggests significantly aged air, consistent with the back trajectory and photochemical aging analyses. The dashed red line is the best fit via orthogonal linear regression. Flight dates, slope and r 2 values are shown for all panels. Full size image Regression of CO against O 3 for all observations ( Supplementary Fig. 2 ) reveals four distinct air mass types observed during CAST and CONTRAST: stratospheric, marine and two distinct polluted regimes, one with elevated CO, NO and O 3 and the other with only elevated CO. Known stratospheric air, characterized by high NO and a strong anti-correlation between CO and O 3 , was encountered on two flights into the subtropics. Data collected during these two flights are excluded from the majority of the HOLW analysis, since our focus is on the tropical troposphere, but are used below to argue against a stratospheric origin of these structures. Parcels with marine characteristics (low CO, NO and O 3 ) all originated from the SH or eastern Pacific ( Fig. 6 ). Back trajectory analysis of the two polluted regimes connects the high CO, NO and O 3 parcels to biomass burning regions in central Africa or Southeast Asia. The high CO/low NO/low O 3 parcels have various geographic origins in Southeast Asia, which could be reflective of emissions of high CO and low NO x from two-stroke engines, dominant in this region of the world. 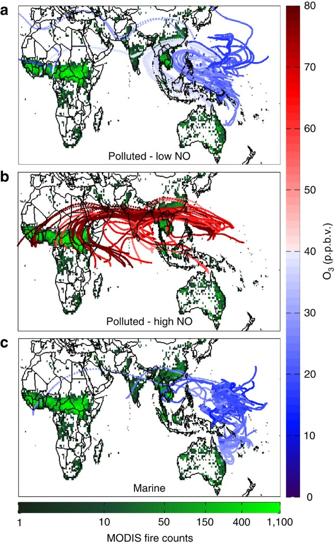Figure 6: Back trajectories by chemical regime. 10-day, HYSPLIT back trajectories for all CAST flights analysed here and CONTRAST RF03–05 and RF07–14 for observed pressures between 300 and 700 hPa. Trajectories are stopped when encountering convective precipitation and coloured by observed O3. Trajectories are separated by the CO regimes illustrated inSupplementary Fig. 2: (a) Polluted—low NO (CO >95 p.p.b.v. and NO <40 p.p.t.v.), (b) Polluted—high NO (CO >95 p.p.b.v. and NO >50 p.p.t.v.), and (c) Marine (CO <80 p.p.b.v. and NO <30 p.p.t.v.). The sum of January and February 2014 MODIS fire counts is shown in green. Figure 6: Back trajectories by chemical regime. 10-day, HYSPLIT back trajectories for all CAST flights analysed here and CONTRAST RF03–05 and RF07–14 for observed pressures between 300 and 700 hPa. Trajectories are stopped when encountering convective precipitation and coloured by observed O 3 . Trajectories are separated by the CO regimes illustrated in Supplementary Fig. 2 : ( a ) Polluted—low NO (CO >95 p.p.b.v. and NO <40 p.p.t.v. ), ( b ) Polluted—high NO (CO >95 p.p.b.v. and NO >50 p.p.t.v. ), and ( c ) Marine (CO <80 p.p.b.v. and NO <30 p.p.t.v.). The sum of January and February 2014 MODIS fire counts is shown in green. Full size image Analysis of other chemical tracers suggests that the observed O 3 in the HOLW structures is likely produced photochemically in biomass burning plumes. Both HCN and CH 3 CN are emitted almost exclusively by biomass burning [36] . Elevated mixing ratios of either species in an air parcel therefore suggests a biomass burning origin. 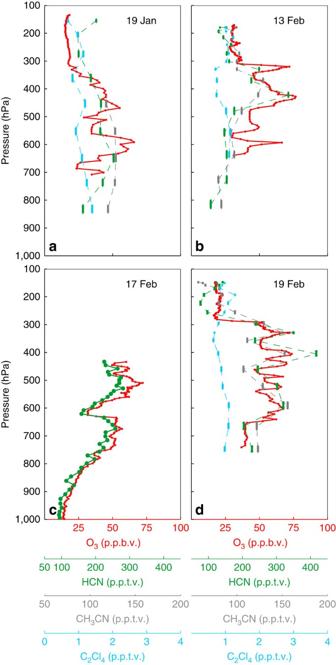Figure 7: Anthropogenic tracers in the HOLW structures. Sample profiles from CONTRAST (a,b,d) and CAST (c) from the four flights shown inFig. 2. O3(red), CH3CN (grey), HCN (green) and C2Cl4(light blue) are shown. O3data are 10 s averages. CH3CN and C2Cl4were not measured during CAST. CONTRAST HCN, CH3CN and C2Cl4were sampled for 35 s at 2 min intervals. CAST HCN was sampled for 30 s. Vertical bars show the pressure range traversed during sampling. Figure 7 shows the profiles of these two species as well as O 3 and the industrial tracer tetrachloroethylene (C 2 Cl 4 ) for the same flights as Fig. 2 . Panels b–d show very tight correlations of O 3 with HCN and CH 3 CN, while, in panel a, HCN and CH 3 CN are elevated between 400 and 700 hPa. Over the entire campaign, air parcels with back trajectories that trace back to Africa and Southeast Asia have a high correlation between O 3 and HCN ( r 2 =0.80), demonstrating significant biomass burning influence. The enhancement ratio of CH 3 CN to CO (4.02 p.p.t.v./p.p.b.v.) for the HOLW structures is consistent with CH 3 CN emissions from tropical forest burning ( Supplementary Fig. 3 ) [37] and is significantly higher than the enhancement ratio for CH 3 CN emissions from fossil fuel combustion (<0.1 p.p.t.v./p.p.b.v.) [38] . The biomass burning tracers benzene (C 6 H 6 ) and ethyne (C 2 H 2 ) also show strong correlation with CO ( r 2 >0.6) as seen in Fig. 8 , further confirming the origin of these air parcels. Figure 7: Anthropogenic tracers in the HOLW structures. Sample profiles from CONTRAST ( a , b , d ) and CAST ( c ) from the four flights shown in Fig. 2 . O 3 (red), CH 3 CN (grey), HCN (green) and C 2 Cl 4 (light blue) are shown. O 3 data are 10 s averages. CH 3 CN and C 2 Cl 4 were not measured during CAST. CONTRAST HCN, CH 3 CN and C 2 Cl 4 were sampled for 35 s at 2 min intervals. CAST HCN was sampled for 30 s. Vertical bars show the pressure range traversed during sampling. 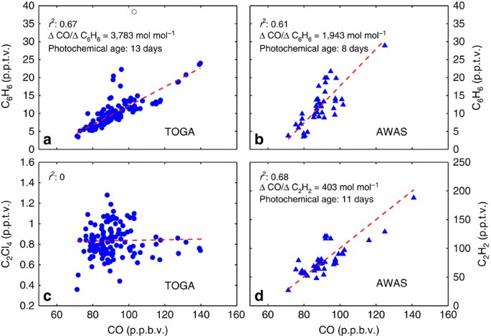Figure 8: Photochemical age of observed air parcels. Regression of CO against: TOGA C6H6(a); AWAS C6H6(b); TOGA C2Cl4(c); and AWAS C2H2(d). Data are only for the HOLW structures (O3>40 p.p.b.v. and RH <20%). The dashed red line is the best fit via orthogonal linear regression. A single data outlier (open circle,a) has been excluded from the analysis. Values ofr2are shown for all panels; enhancement ratios and photochemical ages are shown for panelsa,bandd. Excluding the data point for which C6H6>25 p.p.t.v. for panelbresults in anr2of 0.47, a CO to C6H6enhancement ratio of 1,823 mol mol−1, and a photochemical age of 7 days. Full size image Figure 8: Photochemical age of observed air parcels. Regression of CO against: TOGA C 6 H 6 ( a ); AWAS C 6 H 6 ( b ); TOGA C 2 Cl 4 ( c ); and AWAS C 2 H 2 ( d ). Data are only for the HOLW structures (O 3 >40 p.p.b.v. and RH <20%). The dashed red line is the best fit via orthogonal linear regression. A single data outlier (open circle, a ) has been excluded from the analysis. Values of r 2 are shown for all panels; enhancement ratios and photochemical ages are shown for panels a , b and d . Excluding the data point for which C 6 H 6 >25 p.p.t.v. for panel b results in an r 2 of 0.47, a CO to C 6 H 6 enhancement ratio of 1,823 mol mol −1 , and a photochemical age of 7 days. Full size image Photochemical aging is consistent with the back trajectory analysis. Both C 6 H 6 and C 2 H 2 have lifetimes much shorter than that of CO (ref. 34 ). On the basis of modelled OH from CONTRAST, C 6 H 6 , C 2 H 2 and CO in the TWP have lifetimes of ∼ 6, 12 and 35 days, respectively. All species are primarily removed by reaction with OH, so the change in CO with respect to either C 6 H 6 or C 2 H 2 relative to the initial emissions ratio allows determination of a photochemical age [39] . The photochemical age for C 6 H 6 with respect to CO as determined by the Total Organic Gas Analyzer (TOGA) and Advanced Whole Air Sampler (AWAS) measurements were 13 and 8 days, respectively (see Methods section). The photochemical age for C 2 H 2 was 11 days. These photochemical ages are broadly consistent with the elapsed time between detrainment of biomass burning plumes over Africa and Southeast Asia and transit to the TWP indicated by the back trajectory analysis (5±4 and 7±2 for Southeast Asia and Africa, respectively). The difference between the age indicated by back trajectory analysis and that of photochemical aging is likely due to dilution of biomass burning plumes with ambient air. Dilution would tend to artificially inflate the photochemical age since only CO is present in appreciable amounts in the background TWP. These relatively short values for photochemical age show the composition of air in the HOLW structures is of recent origin. Tagged tracers for biomass burning CO in the CAM-Chem model [40] , run using assimilated meteorology, support our interpretation. A strong African biomass burning influence is frequently seen in the upper troposphere over much of the TWP and extending as far east as Hawaii, at times accounting for 17% of total CO ( Supplementary Fig. 4 ). Deep convection can loft emissions from fires into the upper troposphere, where strong westerlies transport pollutants long distances [41] . Southeast Asian emissions are prominent throughout the tropospheric column ( Supplementary Fig. 4 ). Photochemical ozone production Analysis of ozonesonde observations, CAM-Chem O 3 , and photochemical box model output quantitatively show the high O 3 likely originates within the tropical troposphere. Regions of tropical biomass burning have elevated O 3 as compared with the rest of the tropics, with an O 3 maximum over Africa and the Atlantic basin and a minimum over the TWP [42] . Median O 3 in central Africa and Southeast Asia from CAM-Chem was ∼ 50 p.p.b.v. ( Fig. 9a ) and ∼ 40 p.p.b.v. ( Supplementary Fig. 5a ), respectively, a factor of 2 greater than background O 3 in the TWP. We compare the CAM-Chem output to ozonesonde [43] measurements over Nairobi ( Fig. 9b ) and Hanoi ( Supplementary Fig. 5b ), both strongly influenced by biomass burning, to evaluate CAM-Chem model performance. Mean O 3 from the ozonesondes generally lie within 1σ of the mean CAM-Chem value, suggesting the model accurately captures the O 3 profile in these locations. Means are used because only four or five ozonesonde profiles are available for the study period from each site. Median ozone profiles from CAM-Chem and SHADOZ show comparable agreement in the middle and upper troposphere and substantial differences near the surface ( Supplementary Fig. 6 ). Transport of O 3 from these biomass burning regions cannot explain all of the observed O 3 in the HOLW structures, however, as values frequently peaked at ∼ 75 p.p.b.v., implying there must be photochemical production as the air parcels travel from the biomass burning region. 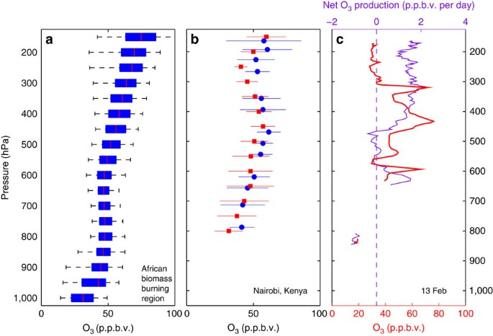Figure 9: Ozone over Africa andin situpotochemical ozone production in the TWP. (a) Vertical distribution of CAM-Chem O3in the African biomass burning region (that is, black boxFig. 4); 5th, 25th, median, 75th and 95th percentiles are shown. (b) Mean ±1σ of SHADOZ ozonesonde observations over Nairobi, Kenya for January and February 2014 (red). Mean ±1σ CAM-Chem O3modelled over Nairobi sampled on the same days as the ozonesondes (blue). (c) O3profile fromFig. 2b(red) and net O3production in the profile (purple, top axis), calculated using the DSMACC photochemical box model (see Methods section). Figure 9: Ozone over Africa and in situ potochemical ozone production in the TWP. ( a ) Vertical distribution of CAM-Chem O 3 in the African biomass burning region (that is, black box Fig. 4 ); 5th, 25th, median, 75th and 95th percentiles are shown. ( b ) Mean ±1σ of SHADOZ ozonesonde observations over Nairobi, Kenya for January and February 2014 (red). Mean ±1σ CAM-Chem O 3 modelled over Nairobi sampled on the same days as the ozonesondes (blue). ( c ) O 3 profile from Fig. 2b (red) and net O 3 production in the profile (purple, top axis), calculated using the DSMACC photochemical box model (see Methods section). Full size image To estimate the net O 3 production in the HOLW structures, a box model constrained by CONTRAST observations (see Methods section) was run for the profiles shown in Fig. 2 . Net O 3 production in the HOLW structures was on the order of ∼ 2 p.p.b.v. per day ( Fig. 9c and Supplementary Fig. 7 ). The value calculated here is a lower bound to net O 3 production in the plume. It is likely that photochemical production along the flight track is significantly lower than in fresh biomass burning plumes, which would be enriched in both NO x and volatile organic compounds (VOCs) as compared with the more aged air observed in CONTRAST. Lightning, a significant contributor to upper-tropospheric NO x (ref. 44 ), would likely further enrich fresh plumes that were lofted into the upper troposphere through deep convection. These fresh plumes can have O 3 production rates of 7 p.p.b.v. per day or higher [42] . As the air ages, however, the abundance of HNO 3 in the plume increases [34] , making NO x unavailable for O 3 production. OH will also oxidize VOCs to less reactive species, and dilution with background air will tend to counteract photochemical O 3 production. Nevertheless, a net O 3 production rate of ∼ 2 p.p.b.v. per day over 5–10 days, combined with initial O 3 of 40–50 p.p.b.v. in the outflow of biomass burning, is consistent with the observed O 3 in the HOLW structures. Low water vapour origin We now turn to the origin of low H 2 O. As with O 3 , H 2 O observed during CAST and CONTRAST has two distinct modes, suggesting that H 2 O in the TWP is controlled both locally and by large-scale processes from outside the study region. For air parcels with HCN <150 p.p.t.v., the H 2 O profile follows the saturation vapour pressure ( Fig. 3b , blue boxes), suggesting that the H 2 O mixing ratio is controlled by local thermodynamics associated with deep convection. CONTRAST flights designed to measure fresh convective outflow were the only tropical flights where HOLW structures were not observed [15] . Parcels with HCN >150 p.p.t.v. had H 2 O mixing ratios an order of magnitude lower than the local saturation vapour pressure. This is consistent with transport of dry air from outside of the TWP. Potential mechanisms to produce the dry air include horizontal advection from the mid-latitudes as well as large-scale descent in the tropics. The association of low H 2 O with high HCN indicates these air parcels originate from biomass burning regions. AIRS measurements [45] and trajectory analysis strongly support our supposition that the observed departures from background H 2 O result from large-scale descent in the tropics. The ascending and descending branches of the Hadley Cell, as determined by AIRS OLR, are shown in Fig. 4c as regions with OLR <250 Wm −2 (blue) and OLR >250 Wm −2 (red), respectively [46] . AIRS H 2 O averaged over the ascending branch agrees well with in situ H 2 O in the low HCN air parcels ( Fig. 3b ). Regression of in situ H 2 O observations from CONTRAST to co-located AIRS retrievals of H 2 O ( Supplementary Fig. 8 ) shows these data sets are in excellent agreement ( r 2 =0.98), allowing for direct comparison of the satellite-retrieved H 2 O to the in situ observations. These profiles are characteristic of deep convection, leading to RH >70%. Back trajectories show the RH <20% air parcels frequently originate in the ascending branch of the Hadley cell, flow anti-cyclonically towards the descending branch, and then reach the TWP along the prevailing westerlies ( Fig. 4 ). Air parcels originating over Africa descend 202±64 hPa, on average, leading to significant decline in RH during transit to the TWP ( Fig. 4b ). Figure 3c shows the AIRS H 2 O profile over Africa (orange lines and squares). The final H 2 O profile over the TWP after subsidence (circles), assuming conservation of the H 2 O mixing ratio in transit, quantitatively agrees with in situ H 2 O for the enhanced HCN mode (grey symbols, Fig. 3b ). Similar agreement is found for AIRS H 2 O profiles over Southeast Asia ( Fig. 3d ). This analysis demonstrates large-scale descent of tropical biomass burning plumes, on their transit to the TWP, can produce the dry element of the HOLW structures. Drying of the air parcels by mixing with mid-latitude air or transport to higher latitudes is not supported by the back trajectory analysis. To determine whether air parcels were moistened or dried during transit, the difference between the trajectory starting point (that is, the trajectory initialization point along the flight track) and the H 2 O mixing ratios at the trajectory end point (that is, 10 days before observation or the point of last precipitating convection) was calculated for all HOLW structures. Water vapour mixing ratios were calculated from the RH and temperature output by the HYSPLIT model along each trajectory. Supplementary Fig. 9 shows a histogram of these changes in H 2 O. For the majority of air parcels (>80%), the H 2 O mixing ratio either increased or did not change in transit to the TWP. This moistening indicates that the majority of the HOLW structures encountered by the CAST and CONTRAST aircraft did not require additional condensation after detrainment to account for the low RH. In fact, these air parcels moistened (experienced a modest increase in H 2 O mixing ratio) in transit, likely due to mixing with background air. The low RH is due to large-scale descent in the tropics and does not require condensation in the mlUT. Potential origins outside the tropical troposphere Mixing with mlUT air is inconsistent with the air mass history and observed composition of the HOLW structures. Parcel trajectories with high O 3 began in the tropics and remained south of the jet core ( Fig. 4a ), indicating minimal contact with mid-latitude air. None of the back trajectories connect the HOLW air parcels to the mid-latitudes. This is consistent with the chemical composition of the filaments. Tetrachloroethylene (C 2 Cl 4 ), a tracer of industrial pollution, has an atmospheric lifetime on the order of 4 months and is primarily emitted in the Northern Hemisphere mid-latitudes, creating a strong latitudinal gradient. Air masses in the tropics influenced by mid-latitude emissions from China frequently have C 2 Cl 4 mixing ratios >2 p.p.t.v. versus a tropical background of 1 p.p.t.v. or less [47] . Tetrachloroethylene mixing ratios in the HOLW structures are a factor of 1.7 times smaller than that observed in the mid-latitude free troposphere during CONTRAST (0.89 and 1.52 p.p.t.v., respectively), suggesting little influence from the mid-latitudes. This is further confirmed by the lack of correlation between C 2 Cl 4 and either high O 3 ( Fig. 7 ) or CO ( Fig. 8c ). Stratospheric origin is also inconsistent with the observed composition of the HOLW structures. Elevated O 3 in the remote TWP can have plausible sources from the polluted troposphere or the O 3 rich stratosphere, resulting in enhancements of a similar magnitude. Mixing line analysis using measurements of at least two other tracers with distinctly different abundances in the troposphere and stratosphere can be used to assess the relative contribution of each potential source [48] . Here we use CO and H 2 O as tracers of the polluted troposphere and the stratosphere, respectively (see Methods section). The mixing line analysis shows that to reproduce the observed H 2 O profile, mixing of stratospheric and background air would require >90% stratospheric air for the majority of observed parcels ( Fig. 10b ) and, in turn, a stratospheric CO mixing ratio of >75 p.p.b.v. for the vast majority of the air parcels (red bars, Fig. 10c ). Observed stratospheric CO was 47.6±6 p.p.b.v. (2σ; grey bar, Fig. 10c ). Only ∼ 1% of parcels had an inferred stratospheric CO within the observed range of stratospheric CO, demonstrating a negligible role for stratospheric influence on the HOLW structures using mixing line analysis. Stratospheric influence was also estimated by interpolating PV to the calculated back trajectories. Only 4% of observed air parcels encountered stratospheric air, defined as intersecting a PV surface >2 PVU (ref. 49 ) along the trajectory ( Fig. 10a ). Relaxing the tropopause definition to 1.5 PVU does not significantly alter this percentage. The combination of low PV air along the trajectories and the mixing line analysis indicates negligible stratospheric influence on the composition of the TWP mid-troposphere during CAST and CONTRAST. 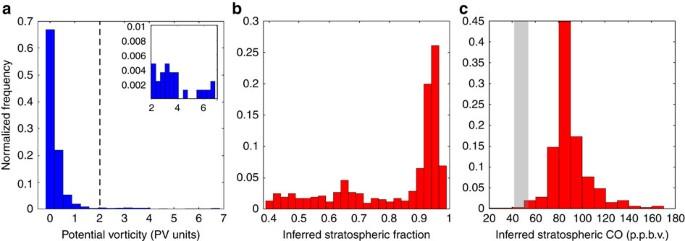Figure 10: Negligible stratospheric influence on the composition of the TWP troposphere. (a) Distribution of the maximum absolute value of PV along the back trajectories for all air parcels observed between 300 and 700 hPa that have travelled over the southeast Asian and/or African biomass burning regions. (b) Distribution of the inferred stratospheric fraction of air (STRAT) needed to explain the low H2O in the HOLW filaments, if the depression in H2O were solely due to stratospheric intrusion. (c) Distribution of inferred stratospheric mixing ratio of CO (COSTRAT INFERRED) assuming the fraction of stratospheric air shown inb. Grey area represents the mean ±2σ of CO observed in the stratosphere during CONTRAST RF15 (O3>200 p.p.b.v.). This mixing line analysis suggests negligible stratospheric influence on the composition of the TWP mid-troposphere during CAST and CONTRAST. Figure 10: Negligible stratospheric influence on the composition of the TWP troposphere. ( a ) Distribution of the maximum absolute value of PV along the back trajectories for all air parcels observed between 300 and 700 hPa that have travelled over the southeast Asian and/or African biomass burning regions. ( b ) Distribution of the inferred stratospheric fraction of air ( STRAT ) needed to explain the low H 2 O in the HOLW filaments, if the depression in H 2 O were solely due to stratospheric intrusion. ( c ) Distribution of inferred stratospheric mixing ratio of CO (CO STRAT INFERRED ) assuming the fraction of stratospheric air shown in b . Grey area represents the mean ±2σ of CO observed in the stratosphere during CONTRAST RF15 (O 3 >200 p.p.b.v.). This mixing line analysis suggests negligible stratospheric influence on the composition of the TWP mid-troposphere during CAST and CONTRAST. Full size image Frequent deep convection in the eastern Pacific likely prevents stratospheric air from reaching the study region. The westerly duct near 180–200° E, a region of preferential transport from the mlUT to the tropics, could potentially supply stratospheric HOLW air to the study area [50] . However, trajectories originating from the SH and eastern Pacific encountered precipitating convection ∼ 2.2 days before observation, that is, these trajectories do not extend back to the westerly duct. Convection promotes mixing with MBL air, removing any extra-tropical signature, as evidenced by the low O 3 mixing ratios for air originating from the eastern Pacific as discussed above. We have shown that the high O 3 in the HOLW structures sampled in the TWP during winter 2014 is quantitatively consistent with a tropical, biomass burning source and that the low H 2 O mixing ratio is consistent with large-scale descent in the tropics. In a sense, low RH acts as a tropospheric age of air indicator in the tropics. Photochemical O 3 production driven by emissions from biomass burning regions, in combination with large-scale descent of tropical, tropospheric air parcels that do not experience active precipitation, leads to a strong anti-correlation of H 2 O and O 3 . Prior analyses of HOLW structures, which suggested an extra-tropical tropospheric origin [12] , [18] , [19] , [20] , [25] , lacked the chemical sophistication of CAST and CONTRAST, relying primarily on ozonesondes or a limited number of chemical tracers in their analyses. Dynamical features suggested as possible mechanisms to bring dry air into the tropics—intrusions of high PV [27] , Rossby wave breaking [26] , and drying through mixing with the subtropical jet [28] , [29] —are inconsistent with the results presented here. These prior studies tend to focus on the subtropics rather than the tropics, use trajectories calculated without consideration of convective precipitation and at times in isentropic coordinates, or provide an interpretation for H 2 O that is qualitative rather than quantitative. Our aircraft and satellite data indicate, in agreement with Dessler and Minschwaner [30] , that large-scale descent in the tropics associated with the Hadley circulation exerts primary control on the H 2 O composition of the TWP troposphere for air parcels that have not experienced recent convection. The attribution of the high O 3 in these HOLW structures suggests a potentially larger role for biomass burning in the radiative forcing of climate in the remote TWP than is commonly appreciated. Tropical tropospheric O 3 is a greenhouse gas, exerting a strong radiative forcing on global climate [2] , [3] . However, present efforts to limit emissions of O 3 precursors are primarily focused on industrial activities and fossil fuel combustion that occur outside the tropics [51] . If the high O 3 in these structures is primarily of tropical origin, then present legislation to limit the emission of O 3 precursors in the extra-tropics may have little, if any, positive impact for the radiative forcing of climate due to tropospheric O 3 . While it is beyond the scope of this paper to estimate the radiative effects of these HOLW structures, biomass burning [52] and HOLW [18] structures are common features of the tropics throughout the year, implying that these structures could have a substantial impact on both global and regional radiative forcing of climate. Field campaigns The CONTRAST campaign consisted of 13 research and 4 transit flights conducted using the National Center for Atmospheric Research (NCAR) Gulfstream V aircraft during January and February 2014. Objectives of the campaign included determining the budget and speciation of very short-lived halogen compounds in the TWP and investigating the transport pathways of these and other chemicals from the MBL to the tropical tropopause layer in a strongly convective environment. Research flights (RF) were either based out of Guam (13.5° N, 144.8° E) or conducted in transit between Broomfield, CO (39.95° N, 105.1° W), the home-base of the Gulfstream V, and Guam. Flights from Guam spanned latitudes from the northern coast of Australia to Japan and altitudes from ∼ 0.5 to 15.5 km. Transit flights (RF01, RF02, RF16 and RF17) as well as flights that sampled primarily mid-latitude air (RF06 and RF15) have been excluded from our analysis, unless otherwise indicated. Tracks of the 11 CONTRAST flights considered here are shown in Fig. 1 ; these flights include all that sampled exclusively in the tropics. In all, 63 vertical profiles were conducted during these flights, offering unprecedented sampling in the middle and upper troposphere of the TWP. RF15 sampled the lower, mid-latitude stratosphere near Japan, as evidenced by O 3 mixing ratios that approached 1 p.p.m.v. The mixing ratio of stratospheric species quoted here are taken from this flight segment, where stratospheric air is defined as having O 3 >200 p.p.b.v.. The NCAR Gulfstream V aircraft was outfitted to measure various trace gases, meteorological parameters and radiative flux. O 3 , NO and NO 2 were measured by chemiluminescence at 1 Hz (ref. 53 ). The 1σ precisions of O 3 , NO and NO 2 at 1 Hz sampling frequency, in the troposphere, are below 0.5 p.p.b.v., 10 p.p.t.v. and 20 p.p.t.v., respectively. Total uncertainties are 5% for NO and O 3 and is 20% for NO 2 . O 3 has been corrected for quenching owing to ambient H 2 O (ref. 54 ). CO was also measured at 1 Hz, with an Aero-Laser 5002 vacuum ultraviolet fluorescence instrument [55] with a 2σ uncertainty of 3 p.p.b.v.±3%. Water vapour was measured by an open path, laser hygrometer at two wavelengths (1,853.37 and 1,854.03 nm), allowing for the sampling of H 2 O mixing ratios spanning 5 orders of magnitude [32] . Data were reported at 1 Hz with a 2σ precision of <3%. RH was calculated from observed H 2 O and temperature. Reported RH is with respect to water for temperatures above 0 °C and with respect to ice for temperatures below 0 °C. Formaldehyde (HCHO), necessary for modelling OH and HO 2 , was measured at high frequency using laser induced by the in situ airborne formaldehyde (ISAF) instrument [56] . HCHO was reported by ISAF at 1 Hz with a 2σ uncertainty of ±20 p.p.t.v.. TOGA measured a suite of trace gases via gas chromatography/quadrupole mass spectrometry with a sampling time of 35 s and 2 min between sampling periods [57] . Measured species relevant to this study are hydrogen cyanide (HCN), acetonitrile (CH 3 CN), tetrachloroethylene (C 2 Cl 4 ), acetone (CH 3 COCH 3 ), acetaldehyde (CH 3 CHO), propane (C 3 H 8 ) and HCHO. AWAS also measured a suite of trace gases, including ethyne (C 2 H 2 ) and benzene (C 6 H 6 ). AWAS acquires up to 60 samples of ambient air per flight in electropolished stainless-steel canisters. Sampling time is pressure dependent. Canisters were analysed post-flight using gas chromatography mass spectrometry. All CONTRAST data used in this study have been averaged over the TOGA observation time, unless otherwise indicated. The sampling resolution for vertical flight segments for data averaged over the TOGA sampling period is ∼ 210 m. Photolysis frequencies were calculated from up and downwelling, spectrally resolved actinic flux density by the HIAPER Airborne Radiation Package (HARP). The system uses independent, 2π steradian optical collectors connected via ultraviolet enhanced fiber optics to charged-coupled device detectors. Spectra were collected every 6 s at ∼ 0.8 nm resolution between 280 and 600 nm with a full-width at half maximum of 1.7 and 2.4 nm in the ultraviolet and visible, respectively. Total photolysis frequencies were calculated from the actinic flux as well as laboratory determinations of molecular cross sections and quantum yields [58] . The CAST campaign was conducted simultaneously with CONTRAST. Whereas observations during CONTRAST were concentrated in the mid- to upper troposphere, the goal of CAST was to observe O 3 , CO, NO, very short-lived organic halogen species and radicals in the MBL and lower troposphere. Together, the two campaigns provide coverage of the TWP from just above the ocean surface to the base of the tropical tropopause layer. CAST flights were based out of Guam, Chuuk (7.4° N, 151.8° E), and Palau (7.5° N, 134.5° E) and covered altitudes from near the surface (30 m above mean sea level) to 8 km. The research portion of this campaign consisted of 23 flights during January and February 2014; 17 of these flights, as shown in Figure 1, provided observations between pressures of 300–700 hPa and are analysed here. CONTRAST and CAST flights were jointly coordinated at a shared operations center in Guam. CAST was conducted using the Facility for Airborne Atmospheric Measurements BAe-146 aircraft. NO was measured with an air quality design, 2-channel chemiluminescence instrument through reaction with O 3 with a 2σ uncertainty of 15%. O 3 was measured at 0.1 Hz with a thermo environmental 49c O 3 analyser by ultraviolet absorption with a 2σ uncertainty of ∼ 0.8 p.p.b.v. CO was measured with an Aero-Laser 5002 instrument at 1 Hz with a 2σ uncertainty of ∼ 1.4 p.p.b.v.. Water vapour mixing ratios were calculated from the observed dew point, measured with a General Eastern dew point hygrometer. HCN was measured by chemical ionization mass spectrometry [59] . No wingtip-to-wingtip comparisons of observations for the CAST and CONTRAST campaign instruments were acquired, due to air traffic concerns in the remote TWP. To compare HCN observations, data from TOGA and the chemical ionization mass spectrometry instrument were selected for background conditions (RH >70% and O 3 <25 p.p.b.v.) and sorted into 0.5 km bins. The mean ±1σ values of HCN for both campaigns strongly overlap, with CAST HCN slightly lower. The mean ratio of CAST to CONTRAST HCN for all altitude bins was 0.90±0.21. A similar process was used to compare O 3 observations, selecting for measurements with RH >70%. The mean CAST to CONTRAST ratio of O 3 values was 0.98±0.26. Since flights were conducted in different air masses and often on different days, this agreement indicates the measurements of O 3 and HCN obtained during CAST and CONTRAST are directly comparable. Sondes Profiles of ozone were measured with electrochemical concentration cell ozonesondes from SHADOZ [43] . Data used here are from observations over Hanoi, Vietnam (21.03° N, 105.85° E) and Nairobi, Kenya (1.28° S, 36.82° E) and were downloaded from the SHADOZ archive ( http://croc.gsfc.nasa.gov/shadoz ). Nairobi data were acquired over 5 days in January and February 2014 using a 0.5% half buffer KI solution with launch times near 8 UTC. Hanoi data were taken over 4 days in January and February 2014, using a 0.5% unbuffered KI solution and launch times near 6 UTC. Satellite data Fire count data are from MODIS onboard the Terra satellite, with a local overpass time of ∼ 10:30 (ref. 52 ). The version 1 monthly product from collection 5, available at a 1 × 1° (latitude, longitude) spatial resolution, is used. MODIS data were downloaded from ftp://neespi.gsfc.nasa.gov . The Level 3, Version 6 daily AIRS product for OLR and water vapour, at 1 × 1° horizontal resolution, is also used [60] , [61] . AIRS is onboard the Aqua satellite with a local overpass time of ∼ 13:30. AIRS data were downloaded from ftp://acdisc.sci.gsfc.nasa.gov/ftp/data/s4pa/Aqua_AIRS_Level3 . Water vapour data cited here are pressure layer averages. Back trajectories Ten day kinematic back trajectories along the flight track were calculated using the NOAA HYSPLIT model [33] . RH, temperature and pressure were output along the trajectory, and H 2 O mixing ratios were calculated using the Clausius–Clapeyron relation. RH, as output by HYSPLIT, is with respect to ice for temperatures below −20 °C and a linear blend of RH with respect to ice and water for temperatures between 0 and −20 °C. HYSPLIT RH was post-processed to convert all points with temperatures between 0 and −20 °C to RH with respect to ice, to render HYSPLIT RH directly comparable to in situ RH. The trajectories allowed for vertical displacement, using estimates of the vertical wind from assimilated meteorological fields. Trajectories from CONTRAST were computed along the flight track at 2 min intervals for pressures between 300 and 700 hPa, corresponding with the time between TOGA observations. CAST data were averaged over 35 s (TOGA integration time) and trajectories were calculated at 2 min intervals (TOGA sampling interval) along the flight track, to make our analysis of CAST data using trajectories analogous to the CONTRAST analysis. Global data assimilation system meteorological fields at 1 × 1° resolution drove the HYSPLIT model. PV, at 6 h resolution from the National Center for Environmental Prediction final analysis, was interpolated to the back trajectory through a bilinear interpolation in the horizontal and a linear interpolation in the vertical and time coordinates. Trajectories were stopped at the point of last precipitating convection. In the TWP, convection promotes mixing with MBL air, altering air parcel composition. Precipitation rates from the tropical rainfall measuring mission satellite were combined with cloud top heights calculated from geostationary satellite infrared measurements. This technique provides coverage of the entire tropics. The convective precipitation product is available at 0.25 × 0.25° (latitude, longitude) resolution with a time step of 3 h. Intersection of a trajectory with precipitating convection was defined as a point on the trajectory being within 25 km of convection in the horizontal and being at or below the cloud top height. The 25 km radius allows for the uncertainty in the back trajectory calculation. CAM-Chem The Community Atmosphere Model version 4.0 (CAM4) is the atmospheric component of the global chemistry-climate model Community Earth System Model [40] . When run with active chemistry, it is known as CAM-Chem. Here the model was run offline, with meteorological fields specified by the NASA GEOS5 model, with a horizontal resolution of 0.94° latitude × 1.25° longitude and 56 vertical levels. The model chemistry scheme includes a detailed representation of tropospheric and stratospheric chemistry ( ∼ 180 species; ∼ 500 chemical reactions), including very short-lived halogens. Fernandez et al . [62] provide details on surface emissions, wet and dry deposition, heterogeneous reactions and photochemical processes of halogens used within CAM-Chem. Anthropogenic emissions are from the RCP 8.5 scenario and biomass burning emissions are from the Fire INventory for NCAR (FINN) [63] . FINN combines observations of biomass burning and vegetation/land cover type from MODIS and emissions factors from multiple data sets to produce a gridded global product with a 1 × 1 km resolution. To determine the relative contributions of biomass burning from individual regions, CO emitted from fires in Africa as well as CO emitted from fires in Southeast Asia were treated as separate variables (referred to as tagged CO in the main paper). Box model Net photochemical production of O 3 was calculated using equation (1) (ref. 31 ) for the CONTRAST profiles shown in Fig. 2 , where brackets indicate concentration and k i represents the rate constant for a given reaction: CH 3 O 2 comprised >95% of RO 2 for the majority of modelled points, so O 3 production from other RO 2 species has been ignored. HO 2 , CH 3 O 2 and O 1 D were not measured; to determine net production of O 3 , these species were calculated using the Dynamically Simple Model of Atmospheric Chemical Complexity (DSMACC) box model [64] . Model runs were only conducted for CONTRAST flights because of lack of necessary VOC data for CAST. The model uses a subset of the Master Chemical Mechanism v3.3 (ref. 65 ) and was initialized with observations of methyl vinyl ketone, methacrolein, acetone, isoprene, methanol and acetaldehyde. NO 2 was estimated using observations of j(NO 2 ), O 3 , NO and modelled values of HO 2 and CH 3 O 2 and then used to initialize the model. The box model was constrained by Gulfstream V observations of meteorological parameters, j(NO 2 ), j(O 1 D), O 3 , CO, NO, HCHO, H 2 O, C 3 H 8 and CH 4 . The abundance of NO and j-values was allowed to vary with time of day. Photolysis frequencies for all reactions were calculated with the Tropospheric Ultraviolet and Visible Radiation model version 4.2 (ref. 66 ) and then scaled using observations of j(O 1 D) and j(NO 2 ). Data were averaged over 10 s. Data from the TOGA instrument were linearly interpolated in time to create a 10 s data set. All output has been integrated over the diel cycle to produce 24 h mean photochemical production of O 3 , because of the diurnal variation of radical species. Model results were compared with output from another box model, the University of Washington Chemical Model (UWCM) [67] , which was constrained and initialized with the same set of input parameters. Between 300 and 700 hPa, the mean ratio of net O 3 production found using DSMACC and UWCM was 1.01. Mixing line analysis Elevated O 3 in the remote TWP can have plausible sources from the polluted troposphere or the O 3 rich stratosphere, imposing enhancements of a similar magnitude. Mixing line analysis using measurements of at least two other tracers with distinctly different abundances in the troposphere and stratosphere can be used to assess the relative contribution of each potential source [48] . Here we use CO and H 2 O as tracers of the polluted troposphere and the stratosphere, respectively. The fraction of stratospheric air, f STRAT was calculated from equation (2), where H 2 O OBS is the observed H 2 O mixing ratio, H 2 O STRAT is the stratospheric H 2 O mixing ratio, and H 2 O TROP is the altitude dependent background tropospheric H 2 O mixing ratio: A constant stratospheric H 2 O mixing ratio of 3 p.p.m.v. was assumed based on the mean observed H 2 O (3.1±0.1 p.p.m.v.) from RF15, which probed the lower stratosphere. Background tropospheric H 2 O was calculated by filtering 10 s averaged data for air parcels with RH >70% and O 3 <20 p.p.b.v., leading to a profile similar to that shown by the blue bars in Fig. 3b . These data were then averaged into 1 km altitude bins. An inferred stratospheric CO mixing ratio, denoted CO STRAT INFERRED was calculated based on f STRAT found using equation (2). The relation for CO STRAT INFERRED is: where variables have analogous definitions to those in equation (2). A value for CO TROP of 85 p.p.b.v. was used, based on the median mixing ratio of CO for air parcels with RH >70%. Since CO TROP showed little variation with altitude, a constant value was used. Photochemical aging Both benzene (C 6 H 6 ) and ethyne (C 2 H 2 ) are tracers of biomass burning pollution and have lifetimes much shorter than that of CO (ref. 34 ). All species are primarily removed by reaction with OH (see reactions 1–5), so the change in CO with respect to either C 6 H 6 or C 2 H 2 , relative to the initial emissions ratio, allows photochemical age to be determined [39] . Rate constants for reactions R3 and R4 are from IUPAC [68] and for reactions R1, R2, and R5 from NASA JPL 2011 (ref. 69 ). All reactions have first-order kinetics, so the ratio of the CO concentration at time t , [CO( t )], to that of benzene, [C 6 H 6 ( t )], is described by equation (4) (ref. 39 ), where k CO is the sum of the rate constants for reactions R1 and R2, k C6H6 is the sum of the rate constants for reactions R3 and R4, ER( t ) is the enhancement ratio of CO to C 6 H 6 at time t , and ER 0 is the ratio of [CO] to [C 6 H 6 ] at the time of emission. The expression for C 2 H 2 is analogous. If all the other variables are known, the expression can be solved for t , the photochemical age. The enhancement ratios of CO to C 6 H 6 and CO to C 2 H 2 over the entire campaign were determined by using an orthogonal linear regression for parcels where O 3 >40 p.p.b.v. and RH <20% ( Fig. 8 ). The slope of these lines is the enhancement ratio. This was done over a campaign-wide basis and not for each profile because of the limited sampling frequency of C 6 H 6 and C 2 H 2 . Separate regressions were done for the TOGA and AWAS C 6 H 6 measurements. Values of r 2 for all regressions were >0.61. The value of ER 0 for the two relations was assumed to be 724 mol CO per mol C 6 H 6 and 241 mol CO per mol C 2 H 2 , which are characteristic of a tropical forest [70] . The photochemical age varied by <0.5 days when emission ratios for other vegetation types [70] were considered. Constant values of temperature (247 K), pressure (350 hPa) and [OH] (1.7 × 10 6 cm −3 ) were assumed when calculating the photochemical age. Temperature and pressure values were the average along the back trajectory for the HOLW filaments, and 1.7 × 10 6 cm −3 is the 24-h mean OH concentration for parcels between 300 and 700 hPa from our box model runs. Equation (4) also assumes that any mixing with ambient air dilutes both species equally. Code availability The CAM-Chem code is available for download at www2.cesm.ucar.edu . An online version of the HYSPLIT model is available at http://ready.arl.noaa.gov/HYSPLIT.php . The DSMACC photochemical box model can be downloaded at http://wiki.seas.harvard.edu/geos-chem/index.php/DSMACC_chemical_box_model and the UWCM box model can be downloaded at https://sites.google.com/site/wolfegm/models . How to cite this article: Anderson, D. C. et al . A pervasive role for biomass burning in tropical high ozone/low water structures. Nat. Commun. 7:10267 doi: 10.1038/ncomms10267 (2016).